Experimental signature of programmable quantum annealing Quantum annealing is a general strategy for solving difficult optimization problems with the aid of quantum adiabatic evolution. Both analytical and numerical evidence suggests that under idealized, closed system conditions, quantum annealing can outperform classical thermalization-based algorithms such as simulated annealing. Current engineered quantum annealing devices have a decoherence timescale which is orders of magnitude shorter than the adiabatic evolution time. Do they effectively perform classical thermalization when coupled to a decohering thermal environment? Here we present an experimental signature which is consistent with quantum annealing, and at the same time inconsistent with classical thermalization. Our experiment uses groups of eight superconducting flux qubits with programmable spin–spin couplings, embedded on a commercially available chip with >100 functional qubits. This suggests that programmable quantum devices, scalable with current superconducting technology, implement quantum annealing with a surprising robustness against noise and imperfections. Many optimization problems can be naturally expressed as the NP-hard problem of finding the ground state, or minimum energy configuration, of an Ising spin glass model [1] , [2] , where the parameters h j and J jk are, respectively, local fields and couplings. The operators are Pauli matrices that assign values {±1} to spin values {↑,↓}. Two algorithmic approaches designed to address this family of problems are directly inspired by different physical processes: classical simulated annealing (SA) and quantum annealing (QA). SA [3] probabilistically explores the spin configuration space by taking into account the relative configuration energies and a time-dependent (fictitious) temperature. The initial temperature is high relative to the system energy scale to induce thermal fluctuations that prevent the system from getting trapped in local minima. As the temperature is lowered, the simulation is driven towards optimal solutions, represented by the global minima of the energy function. In QA [4] , [5] , [6] , [7] , [8] the dynamics are driven by quantum, rather than thermal fluctuations. A system implementing QA [9] , [10] , [11] is described, at the beginning of a computation, by a transverse magnetic field The system is initialized, at low temperature, in the ground state of H trans , an equal superposition of all 2 N computational basis states, the quantum analogue of the initial high-temperature classical state. The final Hamiltonian of the computation is the function to be minimized, H Ising . During the computation, the Hamiltonian is evolved smoothly from H trans to H Ising , where the ‘annealing schedule’ satisfies A (0), B ( T )>0 and A ( T )= B (0)=0. If the change is sufficiently slow and there is no environment, the adiabatic theorem of quantum mechanics predicts that the system will remain in its ground state, and an optimal solution is obtained [12] , [13] . Realistically, one should include the effects of coupling to a thermal environment, that is, consider open system quantum adiabatic evolution [14] , [15] , [16] , [17] , [18] , [19] . An implementation of open system QA has recently been reported in a programmable architecture of superconducting flux qubits [20] , [21] , [22] , [23] , and applied to relatively simple protein folding and number theory problems [24] , [25] . Although quantum tunnelling has already been demonstrated [23] , the decoherence time in this architecture can be three orders of magnitude faster than the computational timescale [23] , [26] , due in part to the constraints imposed by the scalable design. It is interesting to note that this decoherence is in the instantaneous energy eigenbasis (see below). In the circuit model of quantum computation this relatively short decoherence time would imply, without quantum error correction [27] , [28] , that the system dynamics can be described by classical laws [29] . In the context of open system QA, this might lead one to believe that the experimental results should be explained by classical thermalization, or that in essence QA has effectively degraded into SA. Here, we address precisely this question: are the dynamics in open system QA dominated by classical thermalization with respect to the final Hamiltonian, as in SA, or by the energy spectrum of the time-dependent quantum Hamiltonian? We answer this by studying an eight-qubit Hamiltonian representing a simple optimization problem, and show that classical thermalization and QA make opposite predictions about the final measurement statistics. 8-Qubit degenerate Hamiltonian Our Ising Hamiltonian, depicted in Fig. 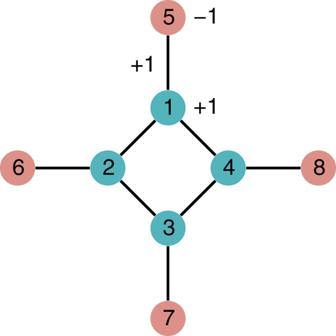Figure 1: Connectivity graph of the degenerate Ising Hamiltonian used in our experiments. The four spins in the central square are the ‘core spins’ (the first four in equations 4 and 5), the four peripheral spins are ‘ancillae spins’ (the last four in equations 4 and 5). As depicted, the local fieldshjof the core spins have value +1 (aquamarine dots), the local fields of the ancillae spins have value −1 (red dots), and all couplingsJjkare ferromagnetic with value +1. A spin inversion (discussed below) would result in different fields and couplings, while relabelling the energy spectrum. 1 , has a 17-fold degenerate ground state Figure 1: Connectivity graph of the degenerate Ising Hamiltonian used in our experiments. The four spins in the central square are the ‘core spins’ (the first four in equations 4 and 5), the four peripheral spins are ‘ancillae spins’ (the last four in equations 4 and 5). As depicted, the local fields h j of the core spins have value +1 (aquamarine dots), the local fields of the ancillae spins have value −1 (red dots), and all couplings J jk are ferromagnetic with value +1. A spin inversion (discussed below) would result in different fields and couplings, while relabelling the energy spectrum. Full size image sixteen of these states form a cluster of solutions connected by single spin-flips of the ancillae spins (equation (4)), while the 17th ground state is isolated from this cluster in the sense that it can be reached only after at least four spin-flips of the core spins (equation (5)). We analyse the spectrum of this Ising Hamiltonian in more detail next. The spectrum can be analysed by first considering the spectrum of the Hamiltonian coupling a single ancilla spin to a core spin (such as spins 5 and 1 in Fig. 1 ). The spectrum, with the core (ancilla) spin written first (second) is the minimum energy is −1 whether the core spin is up or down. Note that if the core spin is up, the minimum energy is −1 whether the ancilla is up or down; this will give rise to a 16-fold degeneracy when we account for all spins below. We analyse the core spins’ energies by first taking into account only their couplings, that is, we analyse the ferromagnetic Hamiltonian of the four central core qubits (spins 1–4 in Fig. 1 ). Denoting by s the number of satisfied couplings (both spins linked by the coupling have the same sign), the energy is 4−2 s , where s ε{0, 2, 4}. The ground states of this Hamiltonian are the configurations |↑↑↑↑› and |↓↓↓↓›. As equation (6) shows that the minimum energy of a core-ancilla pair is −1, when adding the low-energy configurations of the couplings to the ancillae the minimum energy is −8. It also follows from equation (6) that the ground state configurations of the full 8-qubit Hamiltonian are equations (4) and (5). The all-spins down case (5) results from the |↓↓› configuration in equation (6), while the 16-fold degenerate case (4) results from the degeneracy of |↑↑› and|↓↑›. An important feature of the energy landscape of the 8-qubit Hamiltonian is that it does not have any local minima. This can be easily proved by showing that a global minimum can always be reached from any state by performing a sequence of single spin-flips and never raising the energy. To see this, consider an arbitrary state of the system. We can first flip all the ancillae spins to |↓› which, according to equation 6, can be done without raising the energy (independently of the state of the corresponding core spin). Then, we can flip the core spins to satisfy all the couplings between core spins, either making them all |↓› or all |↑›, whichever requires the fewest spin-flips. Again, according to equation 6, this operation will not raise the energy of the core-ancilla pair. Hence, the final state is either the isolated ground state |↓↓↓↓↓↓↓↓› or the state |↑↑↑↑↓↓↓↓› that belongs to the degenerate cluster of ground state configurations. As we show below, classical thermalization predicts that the isolated solution will be found with higher probability than any of the cluster solutions, that is, it is enhanced. Furthermore, after an initial transient, faster thermalization corresponds to a higher probability of finding the isolated solution. Open system QA makes the exact opposite prediction: after an initial transient, the isolated solution is suppressed relative to the cluster, and faster quantum dynamics yields higher suppression (lower probability). Our experimental results are consistent with the open system QA prediction of the suppression effect, and inconsistent with classical thermalization. We next discuss these opposite effects, starting from the classical case. Classical SA predictions Let p i denote the probability of state i in the cluster (4), and p s the probability of the isolated state (5). The probabilities p i are all similar in an ideal implementation, because states in the cluster are connected by single spin-flips, so we consider the average cluster probability . This also helps remove experimental noise and systematic biases that affect the probability of each individual state in the cluster. Enhancement of the isolated state means that p s ≥ p C . Note that the general features of a thermalization process are determined by the spectrum of H Ising and by the combinatorics of state interconversion. As seen above, each of the 17 degenerate ground states can be reached from any other state without ever raising the energy via a sequence of single spin-flips, so that SA never gets trapped in local minima. Consider standard classical thermalization given by single spin-flip transitions whose rate depends only on energy differences (see Methods). The isolated ground state is connected to eight singly excited states via single spin-flips, whereas all states in the cluster are connected via single spin-flips to at most four singly excited states; the other four spin-flips connect between other states in the cluster and hence conserve the energy. During classical annealing at constant low temperature, population feeds faster initially into the isolated state than into any state of the cluster, whence p s ≥ p C . As we report below, our SA numerics show that this is also the case for different cooling schedules throughout the thermalization evolution. Simultaneous double spin-flips do not change this conclusion, and higher order simultaneous spin-flips are less likely physically. In the plots below we used the Metropolis update rule: if Δ E is the energy difference for the update, the transition probability is We have also tested other update rules, such as Glauber’s [30] . The main feature of interest (the isolated state is not suppressed) is unchanged, although the concrete probabilities do depend on the choice of annealing schedule, that is, the functional dependence of the temperature on the number of steps. The SA results for three different annealing schedules are shown in Fig. 2 . The probability p s of the isolated state is always above the average probability p C for a state in the cluster. 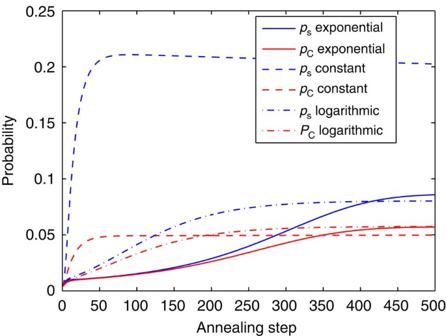Figure 2: SA numerics with different temperature schedules. Probabilities from SA for three different schedules. The probability of the isolated statepsis always higher than the average cluster state probabilitypC. The schedules are: exponential, linearT(n)=Ti/(nrlin+1) and constant temperatureT(n)=0.5, whereTiis the initial temperature,Tfis the final temperature, and,rlin=(Tf/Ti−1)/ntotforntottotal number of annealing steps (seeSupplementary Fig. S1). Figure 2: SA numerics with different temperature schedules. Probabilities from SA for three different schedules. The probability of the isolated state p s is always higher than the average cluster state probability p C . The schedules are: exponential , linear T ( n )= T i /( nr lin +1) and constant temperature T ( n )=0.5, where T i is the initial temperature, T f is the final temperature, and , r lin =( T f / T i −1)/ n tot for n tot total number of annealing steps (see Supplementary Fig. S1 ). Full size image It might be argued that thermalization at constant temperature corresponds most closely to the experimental situation, given that the experimental system remains at an almost constant 17 mK. The corresponding simulation can be seen in Fig. 2 . On the other hand, the energy scale of the Ising model changes during the QA evolution (see the Fig. 4 insert), and the cooling schedule is determined not by the temperature alone but rather by the ratio between the energy scale and the temperature. We also show p s and P C for an exponential schedule with Metropolis updates and different numbers of steps in Fig. 3 . 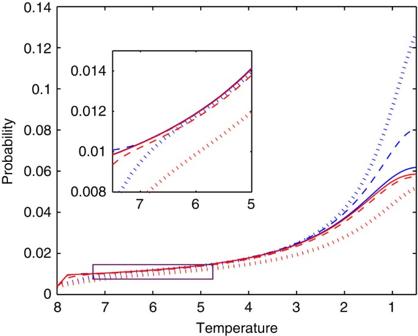Figure 3: SA numerics as a function of annealing speed. Probabilities from SA for varying total numbers of steps. We used the Metropolis update rule with an exponential schedule. The lines correspond to 100 (dotted), 1,000 (dashed) and 10,000 (solid) steps. The upper curves (blue) correspond tops, while the lower curves (red) correspond topC. The inset is a magnification of the boxed part. The separation between the probabilities of the isolated state and the cluster increases as the temperature decreases. Figure 3: SA numerics as a function of annealing speed. Probabilities from SA for varying total numbers of steps. We used the Metropolis update rule with an exponential schedule. The lines correspond to 100 (dotted), 1,000 (dashed) and 10,000 (solid) steps. The upper curves (blue) correspond to p s , while the lower curves (red) correspond to p C . The inset is a magnification of the boxed part. The separation between the probabilities of the isolated state and the cluster increases as the temperature decreases. 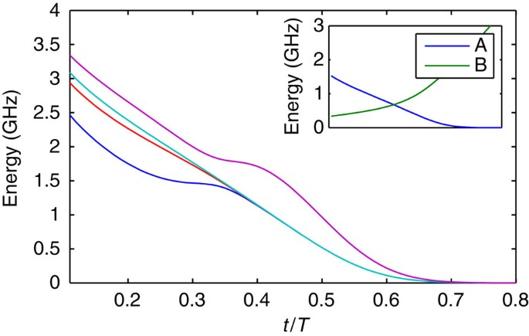Figure 4: Time-dependent gap. We plot the gap between the ground state and the lowest six excited states in the relevant region of the experimental QA evolution. The fourth and fifth excited states are degenerate (that is, the third energy line in the plot corresponds to the gap between a two dimensional subspace and the ground state). After timet=0.5T, the highest energy level shown corresponds to the isolated state with fidelity >0.987. The inset shows the transverse field magnitudeA(t) and Ising Hamiltonian magnitudeB(t) used in our experiments, during the same time interval. Full size image Figure 4: Time-dependent gap. We plot the gap between the ground state and the lowest six excited states in the relevant region of the experimental QA evolution. The fourth and fifth excited states are degenerate (that is, the third energy line in the plot corresponds to the gap between a two dimensional subspace and the ground state). After time t =0.5 T , the highest energy level shown corresponds to the isolated state with fidelity >0.987. The inset shows the transverse field magnitude A ( t ) and Ising Hamiltonian magnitude B ( t ) used in our experiments, during the same time interval. Full size image QA predictions We next analyse the corresponding predictions of QA. A crucial difference with respect to SA is that now the relevant energy spectrum is given by a combination of the final Ising Hamiltonian and the transverse field. Consequently, as shown in Fig. 4 , the degeneracy of the ground space is lifted for times t<T . The isolated state has support only on the highest eigenstate plotted during the second half of the evolution. Given that the system starts in the ground state, the isolated state is suppressed by the energy gap, until this gap vanishes at the end of the evolution. The isolated state remains suppressed nonetheless, as transitions to other low-energy states require at least four spins-flips. The transverse field term, which drives simultaneous spin-flip transitions, is small at large t . If the four spins-flips are not simultaneous, these transitions involve excited states with much higher energy and are suppressed. This predicted QA suppression of the isolated state is confirmed by our closed and open system quantum dynamical simulations (see Fig. 5 ). 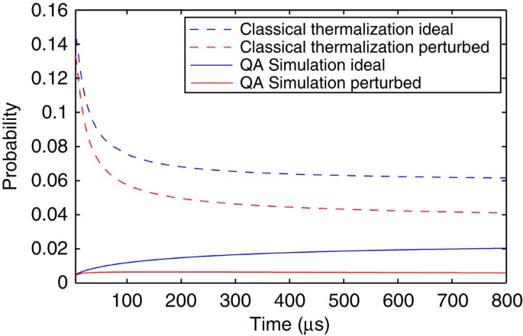Figure 5: Simulations of isolated state suppresion over time. Probability of the isolated state for numerical simulations of classical thermalization (Metropolis update rule) and open system QA as a function of the total annealing timeT. ‘Ideal’ versus ‘perturbed’ corresponds to simulations forHIsingwithout and with a perturbation that increases the energy of the isolated state (red). In classical thermalizationpsalways decreases withT, while it increases for QA in the ideal case. It remains almost constant for QA with the perturbed Hamiltonian. Even if the isolated state is suppressed energetically due to a perturbation ofHIsing, fast classical thermalization can still enhance its probability. The Markovian QA numerical simulations use uncorrelated baths for each qubit, and a single qubitT1~25 ns. A closed system QA simulation predicts zero probability for the isolated state and equal probability for all the states in the cluster (for allT>2 μs). Figure 5: Simulations of isolated state suppresion over time. Probability of the isolated state for numerical simulations of classical thermalization (Metropolis update rule) and open system QA as a function of the total annealing time T . ‘Ideal’ versus ‘perturbed’ corresponds to simulations for H Ising without and with a perturbation that increases the energy of the isolated state (red). In classical thermalization p s always decreases with T , while it increases for QA in the ideal case. It remains almost constant for QA with the perturbed Hamiltonian. Even if the isolated state is suppressed energetically due to a perturbation of H Ising , fast classical thermalization can still enhance its probability. The Markovian QA numerical simulations use uncorrelated baths for each qubit, and a single qubit T 1 ~25 ns. A closed system QA simulation predicts zero probability for the isolated state and equal probability for all the states in the cluster (for all T >2 μs). Full size image We can understand the splitting of the degenerate ground subspace of the Ising Hamiltonian H Ising by treating the transverse field as a perturbation of the Ising Hamiltonian H Ising (thus, treating the QA evolution as that of a closed system evolving backward in time). According to standard degenerate perturbation theory, the perturbation P g of the ground subspace is given by the spectrum of the projection of the perturbation on the ground subspace. Denoting by the projector on the 17-dimensional ground subspace, where ↕ means that the spin can be either up or down, we therefore wish to understand the spectrum of the operator The isolated state is unconnected via single spin-flips to any other state in the ground subspace, so we can write this operator as a direct sum of 0 acting on the isolated state and the projection on the ground subspace of the cluster While σ x acting on any of the four ancillae connects two cluster ground states, σ x acting on any core spin of a cluster state is projected away. Therefore, the perturbation is given by the operator where the sum is over the four ancillae spins. Denoting the eigenbasis of σ x by , with respective eigenvalues ±1, the transverse field splits the ground space of H Ising lowering the energy of |↑↑↑↑++++›, and the four permutations of |−› in the ancillae spins of |↑↑↑↑+++−›. None of these states overlaps with the isolated ground state, which is therefore not a ground state of the perturbed Hamiltonian. Furthermore, after the perturbation, only the sixth excited state overlaps with the isolated state. The isolated state becomes a ground state only at the very end of the evolution (with time going forward), when the perturbation has vanished. Experimental results A diagram of the experimentally achievable coupling configurations is shown in Fig. 6a . The experimental results are shown in Fig. 7 . The key finding that is immediately apparent is that the isolated state is robustly suppressed, in agreement with the QA but not the SA prediction. 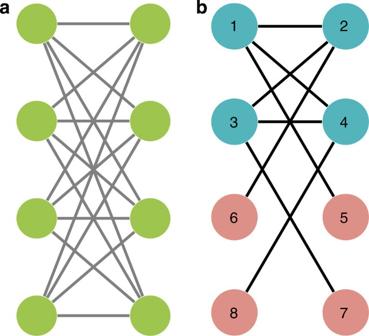Figure 6: Hardware embedding. (a) Schematic depicting the maximal connectivity graph (K4,4) of the qubits inside a unit cell. (b) An embedding ofHIsingfromFig. 1. Different embeddings result in a different assignment of numbers to qubits. Figure 6: Hardware embedding. ( a ) Schematic depicting the maximal connectivity graph ( K 4,4 ) of the qubits inside a unit cell. ( b ) An embedding of H Ising from Fig. 1 . Different embeddings result in a different assignment of numbers to qubits. 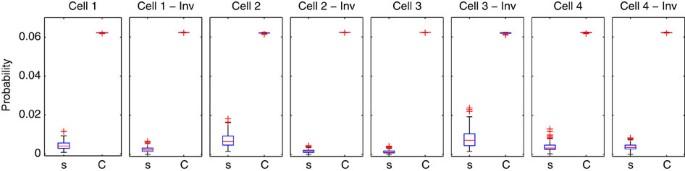Figure 7: Isolated state suppresion for different embeddings. Statistical box plot34of the experimental results forps(left columns) andpC(right columns). The total annealing time wasT=5 μs in each run. In each column the bar is the median, the box corresponds to the lower and upper quartiles, respectively, the segment contains most of the samples, and the +'s are outliers. Cells 1–4 are physically distinct 8-qubit unit cells on the chip. No statistically significant variation is seen as a function of the unit cell number. ‘Inv’ is the case where each local fieldhjis flipped to −hj. In this case the isolated state corresponds to the state |↑↑↑↑↑↑↑↑›, the opposite of equation 5. While this has a small effect for cells 2 and 3, in all cases the isolated state is significantly suppressed, as predicted by QA. This establishes that suppression of the isolated state is not due to a global magnetic field bias. Compare these results with those of the SA numerical simulations inFig. 5. Full size image Figure 7: Isolated state suppresion for different embeddings. Statistical box plot [34] of the experimental results for p s (left columns) and p C (right columns). The total annealing time was T =5 μs in each run. In each column the bar is the median, the box corresponds to the lower and upper quartiles, respectively, the segment contains most of the samples, and the +'s are outliers. Cells 1–4 are physically distinct 8-qubit unit cells on the chip. No statistically significant variation is seen as a function of the unit cell number. ‘Inv’ is the case where each local field h j is flipped to − h j . In this case the isolated state corresponds to the state |↑↑↑↑↑↑↑↑›, the opposite of equation 5. While this has a small effect for cells 2 and 3, in all cases the isolated state is significantly suppressed, as predicted by QA. This establishes that suppression of the isolated state is not due to a global magnetic field bias. Compare these results with those of the SA numerical simulations in Fig. 5 . Full size image Is it possible that suppression has a physical explanation other than QA? The main physical argument along these lines is that a systematic or random bias due to experimental imperfections breaks the 17-fold ground state degeneracy and energetically disfavours the isolated state, thus lowering p s if the system thermalizes. We proceed to examine this and the robustness of the suppression effect. First, note that spin numbers j =1,…,8 must be assigned to the flux qubits before each experimental run. One of the 4!4!2/8=144 possible such ‘embeddings’ allowed by the symmetries of the Hamiltonian and the hardware connectivity graph in each unit cell is shown in Fig. 6b . Second, note that spin inversion transformations commute with H trans , and simply relabel the spectrum of both H Ising and H ( t ): if a certain spin configuration has energy E , then the corresponding spin configuration with the j th spin flipped has the same energy E under . Spin inversions also commute with the spin-flip operations of classical thermalization. Therefore, all of our arguments for the suppression of the isolated state in QA and for its enhancement in classical thermalization are unchanged. Using spin inversions, we can check that the suppression effect is not due to a perturbation of the Hamiltonian such as a magnetic field bias. Indeed, by performing a spin inversion on all eight spins, we obtain a new Ising Hamiltonian where the isolated state is that with all spins-up. If a field bias suppressed the all spins-down state, then it would enhance the all spins-up state. Figure 7 rules this out. We also tested cases with only antiferromagnetic couplings (only ancillae spins are inverted), and with random spin inversions (the set of inverted spins is chosen randomly from a uniform distribution). In all cases we found agreement with the QA prediction, but not with classical thermalization. The results for one such random inversion example are shown in Fig. 8 . 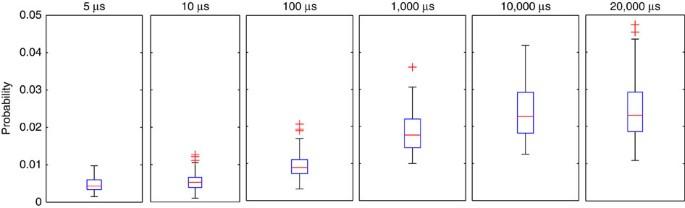Figure 8: Isolated state suppresion over time. Statistical box plot of the probability of the isolated state for a fixed set of qubits, with different annealing times. The Ising Hamiltonianis obtained by inverting spins 2, 3 and 7 ofHIsingfromFig. 1(this particular spin inversion was chosen randomly from a uniform distribution), for thejth of the 144 embeddings. Letdenote the same Hamiltonian after a complete spin inversion. Letv1be a eigenstate ofandv2the inversion ofv1. In this plot, we average the probabilities ofv1andv2for each of the 144 possible embeddings. This compensates for global magnetic field biases (which can be seen inFig. 7, cells 2 and 3). The probability of the isolated state increases with the annealing timeT, in contrast to the classical thermalization prediction. While in classical thermalization an initial distribution concentrated around the cluster can also result in suppression of the isolated state, this suppression is highly unlikely to persist after a random inversion. The experimentally observed increase in probability for the isolated state arises almost entirely from a decreased probability of the cluster (the increase over the range of annealing times shown is ~0.02; only in a few cases an excited state was measured, and never with a probability >0.002). Figure 8: Isolated state suppresion over time. Statistical box plot of the probability of the isolated state for a fixed set of qubits, with different annealing times. The Ising Hamiltonian is obtained by inverting spins 2, 3 and 7 of H Ising from Fig. 1 (this particular spin inversion was chosen randomly from a uniform distribution), for the j th of the 144 embeddings. Let denote the same Hamiltonian after a complete spin inversion. Let v 1 be a eigenstate of and v 2 the inversion of v 1 . In this plot, we average the probabilities of v 1 and v 2 for each of the 144 possible embeddings. This compensates for global magnetic field biases (which can be seen in Fig. 7 , cells 2 and 3). The probability of the isolated state increases with the annealing time T , in contrast to the classical thermalization prediction. While in classical thermalization an initial distribution concentrated around the cluster can also result in suppression of the isolated state, this suppression is highly unlikely to persist after a random inversion. The experimentally observed increase in probability for the isolated state arises almost entirely from a decreased probability of the cluster (the increase over the range of annealing times shown is ~0.02; only in a few cases an excited state was measured, and never with a probability >0.002). Full size image Robust suppression holds even at the level of individual embeddings and spin inversions. We found that p s 3%, while p C <~6% for each of the thousands of such cases we tested (the highest median p s for the experiment in Fig. 7 is 0.004). Thus, suppression survives breaking of the ground state degeneracy, which certainly occurs because of the limited precision of ~10% (ref. 20 ) in our control of { h j , J jk }. The suppression effect is robust because it does not depend on the exact values of these parameters, but on the relatively large Hamming distance between the isolated state and the cluster. Finally, we consider the effect of increasing the annealing time. Open quantum and classical systems converge towards thermal equilibrium. Therefore, if the cause of suppression is the QA spectrum, longer annealing times will result in p s increasing, approaching its Gibbs distribution value. This increase would not be the case if p s were governed by the spectrum of H Ising . In Fig. 5 we compare a numerical simulation of open system QA, using an adiabatic Markovian master equation [19] , with classical thermalization. The quantum prediction of increasing p s is confirmed experimentally, as shown in Fig. 8 . Decoherence basis It is interesting to highlight the difference between decoherence in the instantaneous energy eigenbasis versus the computational basis. We argue that the former is the relevant picture for our experiments. The difference is related, in turn, to whether the master equation is derived in the weak coupling limit (WCL) or singular coupling limit (SCL), the former being the limit where the system Hamiltonian dominates over the system-bath coupling (see Methods). The issue of the basis in which the system decoheres is an important one for QA. In our case the system is initialized to an excellent approximation in the pure ground state of the transverse field . In the computational basis, this corresponds to a density matrix whose elements are all 1/2 N . In the energy eigenbasis, however, only one element of the density matrix is nonzero, corresponding to the lowest energy eigenstate. During an adiabatic evolution, if the decoherence is in the energy eigenbasis, the off-diagonal elements of the density matrix in the energy basis are unimportant and their rapid decay is of no relevance to the final calculation [31] . However, if the decoherence is in the computational basis, the filled density matrix very quickly decoheres to the maximally mixed (infinite temperature) classical state. Therefore, the SCL master equation predicts that the isolated state is not suppressed relative to the cluster of states, which is not in agreement with the experimental results. We thus arrive at our main conclusion: signatures of QA, as opposed to classical thermalization, persist for timescales that are much longer than the single-qubit decoherence time (from 5 μs to 20 ms versus tens of ns) in programmable devices available with present-day superconducting technology. Our experimental results are also consistent with numerical methods that compute quantum statistics, such as Path Integral Monte Carlo (Troyer and Røennow, personal communication). Our study focuses on demonstrating a non-classical signature in experimental QA. Different methods are required to address the question of experimental computational speedups of open system QA relative to optimal classical algorithms. There are no reported experimental measurements of the actual decoherence time for the system that we have considered. Hence, the best we can do at this point is to rely on theoretical estimates or experimental measurements on physical systems that are similar to ours. An estimate of T 2 ~150 ns based on measured features of the noise spectrum has been reported in the literature [32] . There are two experimental reported results, one for a single phase qubit of T 2 ~21 ns (ref. 26 ), and another for a flux qubit of T 2 ~500 ns (ref. 33 ). The estimates thus range from a few tens to several hundred nanoseconds. The important point is that these values do not change our contention that these decoherence times do not destroy the quantum effects present for timescales that are much longer (>5 μs). After the completion of this work, a classical spin dynamics model appeared which also exhibits a suppression of the isolated state [35] . This model can be interpreted as a mean-field model of coherent qubits. The primary purpose of our work has been to compare the predictions of classical simulated annealing to our experimental results and to the predictions of quantum open system dynamics (via the QA master equation), and hence we cannot directly rule out classical spin-dynamics models. However, it is an interesting problem for future study whether classical spin dynamics models can capture the thermalization trend measured experimentally and predicted by the QA master equation ( Fig. 8 ). Experimental system Our experiments were performed using the D-Wave One Rainier chip at the USC Information Sciences Institute, comprising 16 unit cells of eight superconducting flux qubits each, with a total of 108 functional qubits. The couplings are programmable superconducting inductances. The qubits and unit cell, readout, and control have been described in detail elsewhere [20] , [21] , [22] , [23] . The initial energy scale for the transverse field is 10 GHz (the A function in Fig. 4 ), the final energy scale for the Ising Hamiltonian (the B function) is 5.3 GHz, about 15 times the experimental temperature of 17 mK≈0.35 GHz. To gather our data, we ran each of the 144 embeddings 4,000 times, in batches of 1,000 readouts, resetting all the local fields and couplers after each batch. Master equation The SA master equation and the classical thermalization prediction p s ≥ p C can be derived from first principles from an adiabatic quantum master equation [19] . Let H S ( t ) and denote the system and system-bath Hamiltonians. The Lindblad equation is where , {| a ›} is the instantaneous eigenbasis of H S for spin vector a , and . We are interested in the thermalization process in which the density operator is diagonal in the computational basis of spin vectors. The system-bath coupling Hamiltonian then has the form , where σ ± =( σ x ± i σ y )/2. We denote by ( ) the spin vector resulting from flipping the j th spin up (down). From here we arrive at the classical master equation for the populations p a ≡ ρ aa : and the detailed balance condition . Equation 13 is the master equation that we used in our SA numerics. It can also be used to derive the classical thermalization prediction p s ≥ p C . To this end, it can be seen directly that the isolated state is connected to eight excited states with energy −4, giving the rate equation , and also that . Comparing, we conclude that given that initially ps ≥ pc , we always observe ps ≥ pc . A complete derivation is given in the Supplementary Methods . Decay in the energy basis versus the computational basis We demonstrate in detail the difference between decoherence in the energy versus the computational basis. For the analysis in the energy basis it is more convenient to write the system-bath Hamiltonian H SB using Hermitian operators A α and B α . Recall that equation 12 was derived in the WCL. For simplicity, consider the case of non-degenerate energy eigenstates denoted by {| a ›}. Dropping the system Hamiltonian to simplify the notation, the terms that contribute to the population in the instantaneous energy eigenbasis are: where is the transition matrix associated with the transition from the state | a › to the state | b ›, and where we use the shorthand ρ ab =‹ a | ρ ( t )| b › and A ab , α =‹ a | A α | b ›. This result shows that the diagonal elements in the instantaneous energy eigenbasis relax towards the Gibbs distribution. This is crucial as it implies that most of the population will be found in the ground state. The off-diagonal elements of the density matrix in the instantaneous energy eigenbasis are given by: Therefore, we find that the decoherence is described by a system of coupled linear equations involving only the off-diagonal elements of the density matrix. As the Lindblad form of the master equation guarantees complete positivity, the instantaneous eigenvalues of the system of linear equations must be ≤0. The zero eigenvalues correspond to stationary states, which include the instantaneous Gibbs state and any decoherence free subspace. For our case of an independent dephasing model: and γ αβ ( ω )=δ αβ γ( ω ), the latter does not exist. Thus, we find that the off-diagonal elements of the density matrix in the energy eigenbasis decay to zero. As the gap is finite in our system and the single-qubit T 2 is on the order of nanoseconds, this decay occurs on a timescale that is rapid compared with the annealing time. We can contrast the WCL (energy basis) result to the case of the SCL. In this case, the dissipative part of the Lindblad master equation is given by: If we assume that as before, then A α is diagonal in the computational basis, which we denote by {| x ›}, and we choose to work in this basis rather than the instantaneous energy eigenbasis. In this case the dissipative part of the Lindblad master equation for ‹ x | d ρ/ dt | x › vanishes, that is, the populations in the computational basis experience no net thermal excitations and do not equilibrate. For the off-diagonal elements, we obtain an expression similar to equation 15 if we restrict the sums to x ′= x and y ′= y : where A xx ,α =‹ x | A α | x › and ρ xy =‹ x | ρ ( t )| y ›. Thus, here too the density matrix becomes diagonal, but in stark contrast to the case of decoherence in the instantaneous energy eigenbasis, the ground state population is essentially equal to its initial value of 1/2 N . A more detailed derivation of the SCL master equation is presented in Supplementary Methods . How to cite this article: Boixo S. et al. Experimental signature of programmable quantum annealing. Nat. Commun. 4:2067 doi: 10.1038/ncomms3067 (2013).